Recurrent somatic mutation inDROSHAinduces microRNA profile changes in Wilms tumour Wilms tumour (WT) is an embryonal kidney neoplasia for which very few driver genes have been identified. Here we identify DROSHA mutations in 12% of WT samples (26/222) using whole-exome sequencing and targeted sequencing of 10 microRNA (miRNA)-processing genes. A recurrent mutation (E1147K) affecting a metal-binding residue of the RNase IIIb domain is detected in 81% of the DROSHA -mutated tumours. In addition, we identify non-recurrent mutations in other genes of this pathway ( DGCR8 , DICER1 , XPO5 and TARBP2 ). By assessing the miRNA expression pattern of the DROSHA -E1147K-mutated tumours and cell lines expressing this mutation, we determine that this variant leads to a predominant downregulation of a subset of miRNAs. We confirm that the downregulation occurs exclusively in mature miRNAs and not in primary miRNA transcripts, suggesting that the DROSHA E1147K mutation affects processing of primary miRNAs. Our data underscore the pivotal role of the miRNA biogenesis pathway in WT tumorigenesis, particularly the major miRNA-processing gene DROSHA. Wilms tumour (WT) is an embryonal kidney neoplasia that, despite a generally good prognosis, is associated with relapse in up to 15% of cases, requiring additional treatment and leading to adverse long-term effects [1] , [2] . WT affects 1/10,000 children worldwide [3] , [4] and is the most common pediatric kidney cancer. Approximately 10% of WT cases are associated with germline mutations and/or congenital abnormalities, such as those caused by WT1 mutations/deletions (WAGR and Denys–Drash syndromes), 11p15 duplications/imprinting deregulation (Beckwith–Wiedemann syndrome), DIS3L2 mutations (Perlman syndrome), BRCA2 biallelic mutations and the recently described DICER1 mutation in familial pleuropulmonary blastoma syndrome [5] , [6] , [7] , [8] , [9] , [10] . A few genes have been identified as somatically mutated in WT, the most frequent being WT1 , CTNNB1 and WTX , which together account for ~30% of WT cases [11] , [12] , [13] , [14] , [15] . Alterations affecting TP53 , DIS3L2 , FBXW7 , MYCN and DICER1 are also occasionally reported [8] , [16] , [17] , [18] . However, up to 70% of WTs are not associated with an identified somatic mutation, and there is an urgent need to uncover additional mutated pathways for targeting by specific therapeutic agents. In this study, we use whole-exome sequencing (WES) and targeted sequencing of core genes of the microRNA (miRNA) biogenesis pathway to identify somatic mutations in WT. We reveal that DROSHA mutations occur in 12% of WT samples (26/222)—the majority of them in a recurrent hotspot (E1147K); moreover, we identify unique truncating and missense mutations in other miRNA-processing genes ( DGCR8 , DICER1 , XPO5 and TARBP2 ). In addition, we evaluate the miRNA expression pattern of DROSHA -E1147K-mutated tumours and cell lines expressing this mutated protein and determine that the E1147K mutation leads to changes in the miRNA profile, predominantly causing downregulation of a subset of mature miRNAs. Our results provide evidence that DROSHA and the miRNA biogenesis pathway may have a crucial role in WT tumorigenesis. Identification of DROSHA mutations To identify somatic mutations possibly associated with WT tumorigenesis, we performed WES of four samples of a family trio, which included tumour and blood samples from a sporadic WT patient and blood samples from his unaffected parents. 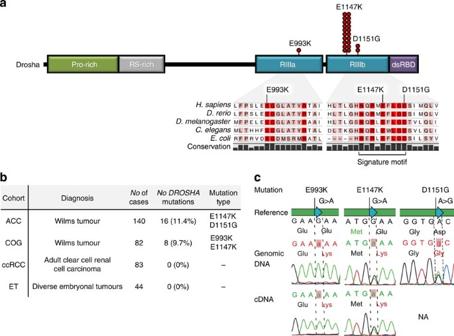Figure 1:DROSHAmutations identified in WTs. (a) Schematic representation of the Drosha protein, showing the position of the three identified mutations in the catalytic RNase III domains (RIIIa and RIIIb). Red circles denote the absolute frequency of each mutation in the entire WT cohort (222 patients). In the magnified region, the missense mutations E993K (RIIIa), E1147K (RIIIb) and D1151G (RIIIb) are shown in the context of RNase III domain conservation across several species; conserved residues are shaded in pink (80% conservation), while invariant residues are in red. The lower bar represents the 9-amino-acid signature motif of RNase III proteins. Domain abbreviations: Pro-rich, proline-rich region; RS-rich, serine/arginine-rich region; RIIIa, RNase IIIa domain; RIIIb, RNase IIIb domain; dsRBD, double-stranded RNA-binding domain. (b) Frequency ofDROSHAmutations (RIIIa and/or RIIIb domains) in the four series of tumours. We investigated two independent WT cohorts (140 from A. C. Camargo (ACC) (including the index case) and 82 from the Children’s Oncology Group (COG)), a group of 83 adult clear-cell renal cell carcinomas (ccRCC), and 44 embryonal tumours from different organs (ET). Mutations in the RIIIa and RIIIb domains ofDROSHAwere detected in ~11% (24/222) of WTs. (c) Sequence traces from DNA (top panels) and cDNA (bottom panels) ofDROSHA-mutated WTs. All tumours harbouring either the E1147K (n=21) or D1151G (n=2) mutation presented the variant in a heterozygous state (DNA and/or RNA data); by contrast, the E993K alteration, which was detected in only one patient, was a homozygous mutation (both tumour DNA and RNA samples). NA, RNA not available. The on-target mean coverage was 67 × , and the percentage of bases covered at least 20 × ranged from 48.3 to 73.4% ( Supplementary Table 1 ). 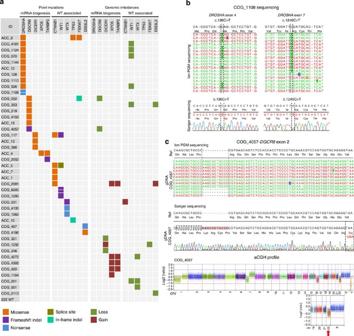Figure 2: Mutation spectrum of WTs. (a) Mutations of the miRNA core processing genes (miRNA biogenesis) and WT-associated genes (WT associated) in 66 fresh-frozen WT samples. Only the genes that were affected by point mutations in at least one sample are shown. Point mutations and indels (left panels) were identified by targeted parallel sequencing, and genomic imbalances (right panels) were detected by aCGH. aCGH data were obtained for 53 samples (2 from ACC and 51 from COG) from a previous study of the group. The coloured squares refer to the corresponding type of point mutation (missense, splice site, frameshift indel, in-frame indel and nonsense) or genomic imbalance (loss and gain). A detailed description of each mutation is provided inTable 1;Supplementary Tables 4 and 5. (b)DROSHAnonsense mutations (c.136C>T; p.Q46* and c.1240C>T; p.R414*) identified in a single patient (COG_1108) by targeted parallel sequencing (upper panels) and validated by capillary Sanger sequencing (bottom panels). (c) Mutations identified in theDGCR8gene. The first panel depicts the 11-nt frameshift duplication identified by targeted parallel sequencing. The middle panel presents the validation by capillary sequencing and the translation of the mutated allele, highlighting the formation of a premature stop codon 62 nt downstream of the alteration. This patient (COG_4057) also presented a heterozygous loss of the entire chromosome 22 (aCGH profile—bottom panel), leading to the deletion of the wild-typeDGCR8allele. Owing to tumour heterogeneity and/or normal cell contamination, this aneuploidy is present in mosaic, resulting in ~30% of reads from Ion Torrent sequencing displaying the wild-type allele and in a log2 ratio value of −0.4 in aCGH analysis. We identified a total of 10 unknown coding somatic variants (5 single nucleotide variants (SNVs) and 5 indel) ( Supplementary Table 2 ). This low rate of somatic alterations was somewhat expected because, in general, embryonal tumours appear to contain few somatic mutations [19] . Of the five identified missense SNVs, only the c.3439G>A (p.E1147K) variant of DROSHA was validated by Sanger sequencing as a somatic mutation that was not present in the blood of the WT patient or his parents (the remaining four variants were not confirmed). DROSHA encodes a nuclear RNase III protein that plays a central role in the miRNA biogenesis pathway. Drosha acts by cleaving primary miRNAs (pri-miRNAs) to release hairpin-shaped pre-miRNAs that are subsequently cut by the cytoplasmic RNase III Dicer to generate mature miRNAs [20] . Drosha possesses two RNase III domains, named RIIIa and RIIIb, which form an intramolecular dimer that cleaves the 3′ and 5′ strands of the stem, respectively [21] , [22] . The DROSHA E1147K mutation identified in this study is a residue of the RIIIb domain that is part of the signature motif of RNase III proteins [21] and that is conserved throughout prokaryotes and eukaryotes ( Fig. 1a ). The affected amino acid is one of four acidic residues that form a metal-binding (Mg 2+ ) cluster at the center of the RNase III catalytic site and thus is essential for catalytic activity [21] . Mutational studies of the Escherichia coli RNASEN protein have demonstrated that amino-acid substitutions of the equivalent residue (E41A in the E. coli protein) abolish the cleavage function of the protein in a Mg 2+ concentration-dependent manner by decreasing the affinity of the protein for metal [23] . The DROSHA E1147K mutation identified in WT leads to the substitution of a negatively charged amino acid (glutamic acid) to a positively charged one (lysine), likely interfering with metal binding at this position. Figure 1: DROSHA mutations identified in WTs. ( a ) Schematic representation of the Drosha protein, showing the position of the three identified mutations in the catalytic RNase III domains (RIIIa and RIIIb). Red circles denote the absolute frequency of each mutation in the entire WT cohort (222 patients). In the magnified region, the missense mutations E993K (RIIIa), E1147K (RIIIb) and D1151G (RIIIb) are shown in the context of RNase III domain conservation across several species; conserved residues are shaded in pink (80% conservation), while invariant residues are in red. The lower bar represents the 9-amino-acid signature motif of RNase III proteins. Domain abbreviations: Pro-rich, proline-rich region; RS-rich, serine/arginine-rich region; RIIIa, RNase IIIa domain; RIIIb, RNase IIIb domain; dsRBD, double-stranded RNA-binding domain. ( b ) Frequency of DROSHA mutations (RIIIa and/or RIIIb domains) in the four series of tumours. We investigated two independent WT cohorts (140 from A. C. Camargo (ACC) (including the index case) and 82 from the Children’s Oncology Group (COG)), a group of 83 adult clear-cell renal cell carcinomas (ccRCC), and 44 embryonal tumours from different organs (ET). Mutations in the RIIIa and RIIIb domains of DROSHA were detected in ~11% (24/222) of WTs. ( c ) Sequence traces from DNA (top panels) and cDNA (bottom panels) of DROSHA -mutated WTs. All tumours harbouring either the E1147K ( n =21) or D1151G ( n =2) mutation presented the variant in a heterozygous state (DNA and/or RNA data); by contrast, the E993K alteration, which was detected in only one patient, was a homozygous mutation (both tumour DNA and RNA samples). NA, RNA not available. 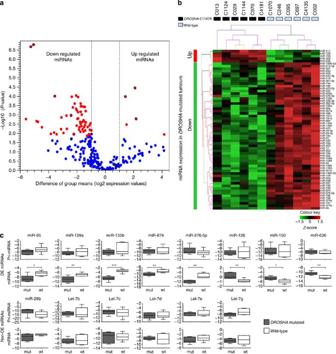Figure 3: Comparison of miRNA expression levels of sixDROSHA-E1147K-mutated and six wild-type WT samples. The samples used in this analysis were fresh-frozen tumours from COG from patients that were not subjected to neoadjuvant chemotherapy. Panelsaandbrefer to the TaqMan Array miRNA profiling experiment. Panelcrefers to the individual TaqMan assays. (a) Volcano plot showing a predominant reduction in mature miRNAs inDROSHA-E1147K tumours. Thexaxis represents the difference of group means (log2 expression values) ofDROSHA-mutated and wild-type tumours; theyaxis represents the statistical significance (−log10P-values). Each miRNA is represented by a dot, and red dots represent those miRNAs that were differentially expressed between the groups; red dots with black borders were selected for pri-miRNA/mature miRNA validation (Fig. 3c). A total of 64 out of 249 miRNAs were differentially expressed between mutated and non-mutated samples. Downregulated miRNAs were over-represented, as 59 miRNAs were downregulated and only 5 were upregulated (Supplementary Table 8). (b) Unsupervised hierarchical clustering analysis based on expression data for the 64 differentially expressed miRNAs confidently discriminatedDROSHA-E1147K from non-mutated samples. (c) Primary and mature miRNA expression. The expression of primary and mature miRNA pairs of eight differentially expressed (DE) and six non-differentially expressed controls (non-DE) was assessed by TaqMan individual assays of the same 12 samples from the array platform. Mean values and s.d. of experiments are shown; statistical significance was calculated using thet-test (*P≤0.01; **P≤0.001; ***P≤0.0001). While all eight DE mature miRNAs were validated as differentially expressed between theDROSHA-mutated and wild-type groups (bottom diagrams), none of the eight DE pri-miRNAs exhibited any significant difference in expression (top diagrams). For the six control miRNAs, no difference in expression level was observed in both mature and pri-miRNAs between the groups (fold changes andP-values are presented inSupplementary Table 9). These results confirm that the differences in mature miRNA expression levels resulted from impaired Drosha activity. Full size image To determine whether the DROSHA E1147K mutation is a recurrent event in WTs, we sequenced the RNase IIIb domain of 139 favourable histology WT samples of all types (14 frozen and 125 formalin-fixed paraffin-embedded (FFPE) tissues) from our Institution (A. C. Camargo Cancer Center—ACC) and 82 frozen favourable histology WT samples, enriched for WTs stages III and IV with a predominant blastema component, obtained from the Children’s Oncology Group (COG) (the clinical features of these cohorts are provided in Supplementary Table 3 ). In addition, we sequenced the entire RIIIa and RIIIb domains of 96 fresh-frozen samples from both cohorts. Overall, ~10% of WTs harboured DROSHA mutations in the investigated domains: 16/140 tumours (11%) from ACC (including the index case) and 8/82 tumours (10%) from COG. The E1147K mutation identified in the index case was a recurrent mutation that was encountered in 20 additional WTs, thus representing 87% (21/24) of DROSHA mutations in the RNase IIIa and b domains. The other three affected patients were positive for a missense mutation in another metal-binding residue of RIIIb (c.3452A>G; p.D1151G—affecting two patients) and a mutation at a residue involved in intramolecular dimerization [21] , [24] of the RIIIa domain (c.2977G>A; p.E993K—affecting one patient) ( Fig. 1a,b ). Interestingly, all E1147K and D1151G mutations were heterozygous, whereas the E993K alteration was a homozygous alteration ( Fig. 1c ) (the likely presence of two mutated alleles was detected by array-comparative genomic hybridization (aCGH) and duplex quantitative PCR (qPCR) [25] — Supplementary Fig. 1 ). Recently, somatic mutations in another miRNA-processing enzyme, Dicer, were identified in WT and other tumours of embryonal/primitive origin (ovarian sex cord–stromal and testicular germ-cell tumours and rhabdomyosarcomas) [18] , [26] . Remarkably, the DICER1 mutations clustered around the four critical metal-binding residues in the RIIIa and, more frequently, RIIIb domain, similar to our findings in DROSHA . To determine whether DROSHA mutations were also present in other embryonal tumours, we sequenced the RNase IIIb domain of 44 samples of 6 different types of embryonal tumours (2 esthesioneuroblastomas, 9 hepatoblastomas, 12 rhabdomyosarcomas and 21 neuroblastic tumours), but no DROSHA mutations were detected in this domain. We also screened 83 adult kidney tumours and did not detect any mutations in this domain ( Fig. 1b ). Targeted sequencing of miRNA-processing genes To investigate the occurrence of mutations in core components of the miRNA-processing pathway in WT, we performed targeted parallel sequencing of 10 genes from this pathway ( DROSHA , DGCR8 , DICER1 , RAN , XPO5 , TARBP2 , AGO1 , AGO2 , GEMIN4 and DDX20 ). To generate a detailed spectrum of somatic mutations in WT, we also included in this targeted sequencing panel 6 genes previously described as mutated in WT ( WT1 , CTNNB1 , WTX , TP53 , DIS3L2 and FBXW7 [8] , [11] , [12] , [13] , [14] , [15] , [16] , [17] , [18] . We evaluated a total of 66 frozen WT samples (15 from ACC and 51 from COG). Figure 2a presents the mutational spectrum of the genes that harboured any point mutations as well as genomic imbalances detected within these genes by aCGH. Figure 2: Mutation spectrum of WTs. ( a ) Mutations of the miRNA core processing genes (miRNA biogenesis) and WT-associated genes (WT associated) in 66 fresh-frozen WT samples. Only the genes that were affected by point mutations in at least one sample are shown. Point mutations and indels (left panels) were identified by targeted parallel sequencing, and genomic imbalances (right panels) were detected by aCGH. aCGH data were obtained for 53 samples (2 from ACC and 51 from COG) from a previous study of the group. The coloured squares refer to the corresponding type of point mutation (missense, splice site, frameshift indel, in-frame indel and nonsense) or genomic imbalance (loss and gain). A detailed description of each mutation is provided in Table 1 ; Supplementary Tables 4 and 5 . ( b ) DROSHA nonsense mutations (c.136C>T; p.Q46* and c.1240C>T; p.R414*) identified in a single patient (COG_1108) by targeted parallel sequencing (upper panels) and validated by capillary Sanger sequencing (bottom panels). ( c ) Mutations identified in the DGCR8 gene. The first panel depicts the 11-nt frameshift duplication identified by targeted parallel sequencing. The middle panel presents the validation by capillary sequencing and the translation of the mutated allele, highlighting the formation of a premature stop codon 62 nt downstream of the alteration. This patient (COG_4057) also presented a heterozygous loss of the entire chromosome 22 (aCGH profile—bottom panel), leading to the deletion of the wild-type DGCR8 allele. Owing to tumour heterogeneity and/or normal cell contamination, this aneuploidy is present in mosaic, resulting in ~30% of reads from Ion Torrent sequencing displaying the wild-type allele and in a log2 ratio value of −0.4 in aCGH analysis. Full size image Point mutations were identified in five miRNA-processing genes ( DROSHA , DGCR8 , DICER1 , XPO5 and TARBP2 ) and in all 6 genes previously associated with WT ( WT1 , CTNNB1 , WTX , TP53 , DIS3L2 and FBXW7). Descriptions of the variants and the clinical data for the patients with mutations are provided in Table 1 and Supplementary Tables 4 and 5 . Interestingly, in 33% (22/66) of WTs, we detected potentially deleterious mutations in genes of the miRNA-processing pathway, while genes previously described to be mutated in WT were detected in 22.7% (15/66) of WTs. We considered as possibly disease-associated all indels, nonsense and splice site mutations, and missense alterations classified as damaging by at least one of the prediction software used ( Fig. 2a ; Table 1 ). The substantial frequency of mutations in genes involved in miRNA biogenesis suggests that impaired miRNA maturation might play a pivotal role in WT. Table 1 Classification of point mutations detected in 66 frozen WT samples. Full size table Among the miRNA-processing genes, DROSHA was most frequently mutated. In addition to the missense mutations previously identified by sequencing the RIIIa and b domains, one missense (c.631C>A; p.P211T) and two novel nonsense mutations (c.136C>T; p.Q46* and c.1240C>T; p.R414*) were identified in this gene. Both nonsense mutations were present in the same patient (COG_1108— Fig. 2b ). Sequencing of allele-specific PCR products amplified from complementary DNA (cDNA) confirmed that each mutation is present in one allele (biallelic mutations) ( Supplementary Fig. 2 ); however, the unavailability of normal tissue from this patient prevented the determination of the nature (somatic or germline) of both mutations. In summary, a total of 6 distinct DROSHA pathogenic mutations were identified in 26 WT samples ( Supplementary Table 6 ). Remarkably, we detected an overlap between the DROSHA point mutations and WT1 genomic losses. Of 10 patients harbouring DROSHA mutations, four also presented loss of the WT1 gene (40%), while the rate of WT1 loss in the whole series was 9% (6/66) ( Fig. 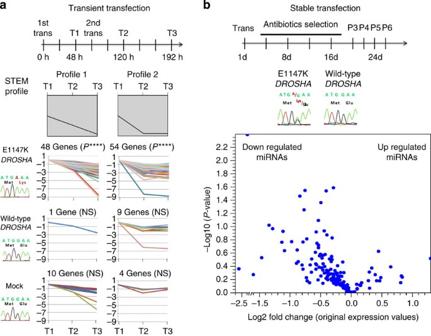Figure 4: miRNA profile in cell line models expressing E1147K Drosha. (a) Time course experiment of miRNA expression in HEK293 cells transiently expressing wild-type or E1147K Drosha. A schematic representation of the experiment is depicted in the top panel: transfections were performed twice in a 72-h interval (1st trans and 2nd trans), and miRNA expression levels were measured at three time points using the TaqMan Array platform (T1, T2 and T3). The middle panel represents the Short Time-series Expression Miner (STEM) analysis profiles, which were used to cluster and analyse the expression data. Of the six considered profiles produced by STEM analysis (Supplementary Fig. 6), E1147K-transfected cells presented two statistically significant profiles—(profile 1:P=2 × 10−16; and profile 2:P=2 × 10−8) that harboured more genes than expected by chance (48 and 54 genes, respectively). These two profiles represent a reduction in mature miRNA levels from time points T1 to T3. ****P≤0.00001. NS, not significant. (b) miRNA expression in HEK293T cells stably transfected with wild-type or E1147K Drosha. The top panel depicts a schematic representation of the experiment, showing the time length of selection and the passages at which cell extracts were collected for miRNA expression analysis. Four passages of each stable cell line were evaluated for miRNA expression using the TaqMan Array platform, and the mean expression values of each miRNA in E1147K and wild-type cells were compared. The middle panel presents the cDNA sequencing traces, which demonstrate that stable transfection resulted in similar expression levels of the mutant and endogenous wild-type alleles. The lower panel displays a volcano plot showing a trend to preferential reduction in mature miRNAs in E1147K-stably transfected cells, characterized by the enrichment of miRNAs species in the left side of the volcano plot. Thexaxis represents the log2fold change between HEK293T-E1147K and wild-type cells; theyaxis represents the statistical significance (−log10P-values). 2a ; Supplementary Table 4 ). We also identified deleterious frameshift mutations in two other miRNA-processing genes: DGCR8 (p.R32fs) and TARBP2 (p.R353fs). DGCR8 together with Drosha forms the microprocessor unit responsible for cleaving pri-miRNAs into pre-miRNAs [22] , [27] , while TRBP (encoded by TARBP2) , together with Dicer, forms the complex necessary for converting pre-miRNAs into mature miRNAs [28] . Remarkably, the patient presenting the frameshift duplication in DGCR8 also harboured a heterozygous loss of the entire chromosome 22, where this gene is located, leading to the deletion of the normal allele ( Fig. 2c ). In addition, non-recurrent missense mutations were identified in DGCR8 (G55S, S92R, E518K, A558T and Y721H), DICER1 (Q48E, I85M and D1810N), XPO5 (V832I) and TARBP2 (R296H). With the exception of the DICER1 D1810N variant located in the RIIIb domain, which was previously described as a driver mutation in other tumour types [26] , the true significance of the remaining missense alterations in WT onset has yet to be revealed. Analysis of miRNA expression profiles The most frequently occurring mutation identified in our study was the DROSHA E1147K mutation (21/222 samples). To elucidate the influence of this mutation on the miRNA maturation process, we compared the mature miRNA expression profile of six DROSHA -E1147K WT samples with six wild-type WTs (without mutations in the miRNA core genes) using a TaqMan Array platform ( Supplementary Table 7 ). Unsupervised assessment of global miRNA expression by principal component analysis revealed that DROSHA -mutated and non-mutated tumours were perfectly discriminated ( Supplementary Fig. 3 ), revealing a strong relationship between the miRNA profile and the presence of the E1147K mutation. Next, we compared the expression levels of miRNAs between the two groups. A total of 64 mature miRNAs were differentially expressed in E1147K-mutated tumour samples compared with wild-type WT, with a predominance of reduced miRNA expression, as 59 miRNAs were downregulated and only 5 were upregulated (fold change ⩾ |2|; false discovery rate (FDR)-corrected P ≤0.05) ( Fig. 3a ; Supplementary Table 8 ). For the 21 miRNAs presenting 5p- and 3p-derived miRNAs in the assay (7 differentially expressed and 15 non-differentially expressed), concordant expression data were detected for both 5p and 3p mature miRNAs ( Supplementary Table 9 ), underscored by similar fold changes for 5p and 3p paired miRNAs. This suggests that in contrast to what is observed for DICER1 mutations affecting the RIIIb domain, which result in a complete absence of 5p-derived miRNAs but have no effect on 3p-derived specimens [29] , the DROSHA E1147K mutation affects miRNAs derived from both strands. Figure 3: Comparison of miRNA expression levels of six DROSHA -E1147K-mutated and six wild-type WT samples. The samples used in this analysis were fresh-frozen tumours from COG from patients that were not subjected to neoadjuvant chemotherapy. Panels a and b refer to the TaqMan Array miRNA profiling experiment. Panel c refers to the individual TaqMan assays. ( a ) Volcano plot showing a predominant reduction in mature miRNAs in DROSHA -E1147K tumours. The x axis represents the difference of group means (log2 expression values) of DROSHA -mutated and wild-type tumours; the y axis represents the statistical significance (−log10 P -values). Each miRNA is represented by a dot, and red dots represent those miRNAs that were differentially expressed between the groups; red dots with black borders were selected for pri-miRNA/mature miRNA validation ( Fig. 3c ). A total of 64 out of 249 miRNAs were differentially expressed between mutated and non-mutated samples. Downregulated miRNAs were over-represented, as 59 miRNAs were downregulated and only 5 were upregulated ( Supplementary Table 8 ). ( b ) Unsupervised hierarchical clustering analysis based on expression data for the 64 differentially expressed miRNAs confidently discriminated DROSHA -E1147K from non-mutated samples. ( c ) Primary and mature miRNA expression. The expression of primary and mature miRNA pairs of eight differentially expressed (DE) and six non-differentially expressed controls (non-DE) was assessed by TaqMan individual assays of the same 12 samples from the array platform. Mean values and s.d. of experiments are shown; statistical significance was calculated using the t -test (* P ≤0.01; ** P ≤0.001; *** P ≤0.0001). While all eight DE mature miRNAs were validated as differentially expressed between the DROSHA -mutated and wild-type groups (bottom diagrams), none of the eight DE pri-miRNAs exhibited any significant difference in expression (top diagrams). For the six control miRNAs, no difference in expression level was observed in both mature and pri-miRNAs between the groups (fold changes and P -values are presented in Supplementary Table 9 ). These results confirm that the differences in mature miRNA expression levels resulted from impaired Drosha activity. Full size image The 64 differentially expressed miRNAs affected by the DROSHA E1147K mutation were used for unsupervised hierarchical clustering of the six E1147K-mutated tumours and six controls (wild-type for the miRNA core genes). The resulting cluster completely discriminated E1147K-mutated from non-mutated WT samples ( Fig. 3b ). Moreover, we also interrogated the expression profile of this set of miRNAs in three additional WT samples with other mutations in the DROSHA or DGCR8 genes (COG_1110: DROSHA homozygous E993K; COG_1108: two nonsense mutations in DROSHA —Q46* and R414*; and COG_4057: DGCR8 frameshift and genomic loss). Interestingly, the two tumours with double hits (COG_1108 and COG_4057) exhibited remarkably lower expression of the affected miRNAs ( Supplementary Fig. 4 ). To determine whether these differences in mature miRNA quantities resulted from impaired activity of DROSHA E1147K in cleaving pri-miRNAs, we evaluated the expression of pri-miRNAs and their matching mature miRNAs ( Fig. 3c ; Supplementary Table 10 ). We selected 8 miRNAs from the 64 miRNAs that were differentially expressed between mutated and non-mutated tumours and six of the 185 miRNAs that did not exhibit significant differences in expression as negative controls. As expected, none of the eight selected pri-miRNA transcripts were significantly differentially expressed between the DROSHA -E1147K and wild-type groups, suggesting no alteration in terms of the transcriptional regulation of these transcripts. By contrast, the differential expression of the corresponding mature miRNAs between the two groups was confirmed, suggesting that these differences were indeed a consequence of defective Drosha processing. No differences in the expression levels of the six miRNAs used as negative controls, whether mature or pri-miRNAs, were observed between the DROSHA -E1147K and wild-type groups. In vitro effects of E1147K DROSHA mutation Next, we used a controlled cell line assay to evaluate the effects of the E1147K mutation on miRNA regulation. We assessed the miRNA expression profile of HEK293 cells transiently transfected with wild-type or E1147K- DROSHA plasmids in a time course experiment to monitor changes in miRNA expression over time. The time course experiment was designed to permit the repopulation of miRNA by action of the mutated protein in the processing of pri-miRNAs to mature specimens. Consistent with our observations in the tumour cohort, E1147K-transfected cells exhibited a significant reduction in mature miRNA levels over time compared with both wild-type DROSHA and mock-transfected cells ( Fig. 4a ; Supplementary Figs 5 and 6 ). Furthermore, 31/59 miRNAs that were downregulated in the DROSHA -mutated tumours also exhibited decreased expression in E1147K-HEK293 transient cells ( Supplementary Table 11 ). Figure 4: miRNA profile in cell line models expressing E1147K Drosha. ( a ) Time course experiment of miRNA expression in HEK293 cells transiently expressing wild-type or E1147K Drosha. A schematic representation of the experiment is depicted in the top panel: transfections were performed twice in a 72-h interval (1st trans and 2nd trans), and miRNA expression levels were measured at three time points using the TaqMan Array platform (T1, T2 and T3). The middle panel represents the Short Time-series Expression Miner (STEM) analysis profiles, which were used to cluster and analyse the expression data. Of the six considered profiles produced by STEM analysis ( Supplementary Fig. 6 ), E1147K-transfected cells presented two statistically significant profiles—(profile 1: P =2 × 10 −16 ; and profile 2: P =2 × 10 −8 ) that harboured more genes than expected by chance (48 and 54 genes, respectively). These two profiles represent a reduction in mature miRNA levels from time points T1 to T3. **** P ≤0.00001. NS, not significant. ( b ) miRNA expression in HEK293T cells stably transfected with wild-type or E1147K Drosha. The top panel depicts a schematic representation of the experiment, showing the time length of selection and the passages at which cell extracts were collected for miRNA expression analysis. Four passages of each stable cell line were evaluated for miRNA expression using the TaqMan Array platform, and the mean expression values of each miRNA in E1147K and wild-type cells were compared. The middle panel presents the cDNA sequencing traces, which demonstrate that stable transfection resulted in similar expression levels of the mutant and endogenous wild-type alleles. The lower panel displays a volcano plot showing a trend to preferential reduction in mature miRNAs in E1147K-stably transfected cells, characterized by the enrichment of miRNAs species in the left side of the volcano plot. The x axis represents the log 2 fold change between HEK293T-E1147K and wild-type cells; the y axis represents the statistical significance (−log10 P -values). Full size image To further validate the effects of the E1147K mutation, we simulated in vitro the heterozygous expression of the mutation observed in the tumours by stably transfecting HEK293T cells with wild-type or E1147K- DROSHA. Stable transfection resulted in reduced expression of the exogenous gene, and cDNA sequencing revealed that both the mutated and endogenous wild-type alleles were expressed in similar levels ( Fig. 4b ; Supplementary Fig. 7 ). Analysis of the miRNA expression profiles demonstrated that E1147K-stably transfected cells also presented a trend to preferential reduction in mature miRNA levels compared with wild-type DROSHA , as demonstrated by the enrichment of miRNAs species in the left side of the volcano plot ( Fig. 4b ). However, as expected, the miRNA downregulation was surely less robust than that observed in tumours or the transient transfection assay, since by using the same arbitrary stringent criteria applied for the tumours (fold change ⩾ |2|; FDR-corrected P ≤0.05) no miRNAs could be classified as differentially expressed between E1147K-stably transfected cells and wild-type. In this study, we identified and characterized the effects of recurrent DROSHA E1147K mutations in WTs. Overall, our data suggest that the predominant effect of DROSHA mutations is the reduction in mature miRNA expression. Drosha and Dicer function in a stepwise manner to generate mature miRNAs. Mutations that abolish the cleavage function of one domain of RNase III proteins with two RIII domains, such as Drosha and Dicer, do not affect the cleavage of the other domain, consequently leading to the formation of incompletely processed RNA substrates [22] , [30] . Given that Dicer most efficiently cuts pre-miRNAs presenting the canonical structure of a two-nucleotide 3′ overhang [31] , the double-stranded RNA structures derived from the defective processing of a mutated Drosha would most likely be unrecognizable by Dicer. Thus, given that amino-acid substitutions in any of the four critical metal-binding residues of Drosha, such as the E1147K mutation, abolish the RNase III catalytic activity of the affected domain, and based on the data observed in our study, we can suggest that pri-miRNAs are incompletely cleaved by the E1147K mutant Drosha, thereby impairing Dicer recognition and ultimately leading to a decreased amount of mature miRNA molecules. We and others have demonstrated that nephrogenesis and Wilms tumorigenesis share gene expression regulation patterns [32] , [33] , [34] , [35] . Furthermore, repression of miRNA maturation through inhibition of DROSHA and DICER1 expression impairs accurate kidney differentiation [36] , [37] , [38] and promotes tumorigenesis in several cell lines [39] . In this context, we speculate that the reduction in mature miRNAs caused by DROSHA E1147K mutations might impair kidney differentiation and contribute to WT onset. In summary, we have demonstrated that the DROSHA E1147K is a recurrent mutation and that DROSHA and other miRNA-processing genes are mutated in about 33% (22/66) of WT samples, implying that defective miRNA biogenesis may contribute to WT development. However, as the COG cohort displays WT samples of predominant blastemal histology, the frequency of mutations in this pathway in a broad unbiased WT series still remains to be determined. Our findings, together with the recent discovery of DICER1 mutations in other tumours [18] , [26] , reveal that mutations disrupting the miRNA-processing machinery represent key events in embryonal tumorigenesis. These insights open a new field of investigation into these neoplasias and highlight this pathway as a putative target for drug development and cancer therapy. Samples Four samples from a family trio were subjected to WES: tumour and blood from one patient (ID=ACC_12) affected by a favourable-histology WT (wild type for WT1 gene) and blood from the unaffected parents. For DROSHA mutation screening, 139 WT samples were retrieved from the Biobank and archives of A. C. Camargo Cancer Center (14 fresh-frozen samples and 125 FFPE samples). The validation cohort comprised 82 WT samples from patients enrolled in the National Wilms Tumour Study (NWTS-5—USA) from the COG (these samples are enriched for WTs stages III and IV with a predominant blastema component, which were selected for a previous gene expression study of our group [40] ). Clinical features of these WT cohorts are described in Supplementary Table 3 . In addition, 44 fresh-frozen samples of six different types of embryonal tumours (2 esthesioneuroblastomas, 9 hepatoblastomas, 12 rhabdomyosarcomas and 21 neuroblastic tumours) and 83 adult kidney tumours (clear-cell renal cell carcinoma) were retrieved from the biobank of A. C. Camargo Cancer Center and were screened for DROSHA mutations. For miRNA global expression evaluation, only RNA from fresh-frozen samples that were not submitted to chemotherapy before surgery was used (samples from COG) (clinical features of samples used in this analysis are described in Supplementary Table 5 ). aCGH data were obtained from a previous study of the group (Krepischi et al ., unpublished data) that investigated genomic gains and losses in a subset of the fresh-frozen samples (2 from ACC and 51 from COG). All samples were obtained with informed consent. This work was conducted in accordance with the principles of the Declaration of Helsinki and was approved by the A. C. Camargo Cancer Center ethics committee under number CEP 764/06. DNA and RNA isolation Genomic DNA and RNA samples were obtained from the DNA and RNA laboratory of A. C. Camargo Biobank. DNA from blood samples was purified using the Puregene Genomic DNA Isolation Kit (Gentra Systems), according to the manufacturer’s instructions. Genomic DNA was obtained from fresh-frozen or FFPE tumours using a phenol:chlorophorm method. RNA was isolated from frozen tumour tissue (10–100 mg) or cell pellets (10 6 cells) using TRIzol (Invitrogen) and Precellys 24 tissue homogenizer (Bertin Technologies). DNA and RNA concentration, purity and integrity were assessed by spectrophotometry (Nanodrop 2000) and microfluidics-based electrophoresis (Agilent 2100 Bioanalyzer), respectively. Supplementary Table 5 presents the RNA integrity (RIN) data of samples used in miRNA and mRNA array experiments. WES WES was performed using the SureSelect 50 Mb All Exons kit (Agilent Technologies), followed by sequencing of 110 base pairs of paired-end libraries in a Solid 5500XL System (Life Technologies). The resulting sequences were mapped to the reference genome (GRCh37/hg19) obtained from UCSC Genome Browser ( http://genome.ucsc.edu ) with Bioscope ( http://www.lifescopecloud.com/ ) and NovoalignCS ( http://novocraft.com/ ). Sequence variants (SNVs and indels) were identified with SAMtools ( http://samtools.sourceforge.net/ ) and the mpileup ( http://samtools.sourceforge.net/mpileup.shtml ) and annotated if present on dbSNP (release #137) or COSMIC v60. Next, the identified variants were considered as possible candidates if base coverage was ⩾ 10 × and variant base was present in at least 15% of the reads, and was not reported in dbSNP. Sanger sequencing and pyrosequencing Fresh-frozen tumours were screened by Sanger sequencing of either genomic DNA or cDNA, while FFPE samples were screened by pyrosequencing of genomic DNA. Sanger PCR was performed with GoTaq Green Master Mix (Promega), purified with ExoSAP-IT (USB Corporation) and sequenced in both directions using an ABI 3130xl DNA sequencer (Life Technologies). The resulting sequences were aligned using CLCBio Genomics Workbench Software (CLCBio). Pyrosequencing PCR was performed with a PyroMark PCR kit (Qiagen), and the PCR products were sequenced according to the manufacturer’s protocol with a PyroMark Q96 ID instrument (Qiagen). The primer sequences used in these analyses are described in Supplementary Table 12 . Mutations identified by Sanger and pyrosequencing were evaluated regarding the conservation of the affected amino acid across several species. RNASE III protein sequences from Homo sapiens (NP_037367.3), Danio rerio (NP_001103942.1), Drosophila melanogaster (NP_477436.1), Caenorhabditis elegans (AAD45518.1) and E. coli (YP_490795.1) were aligned using CLCBio Genomics Workbench Software (CLCBio) ( Fig. 1a ). Gene panel parallel sequencing We designed an Ion AmpliSeq panel using the Ion AmpliSeq Designer v3.0.1 (Life Technologies). The panel was composed of 16 genes: 10 core genes of the miRNA-processing pathway ( DROSHA , DGCR8 , RAN , XPO5 , DICER1 , TARBP2 , AGO1 , AGO2 , GEMIN4 and DDX20 ) and 6 genes previously reported as somatically mutated in WT ( WT1 , CTNNB1 , WTX , TP53 , DIS3L2 and FBXW7 (refs 8 , 11 , 12 , 13 , 14 , 15 , 16 , 17 , 18 ), corresponding to a total of 59.81 kb. Libraries were prepared for 66 fresh-frozen samples using 20 ng of DNA from each sample according to the Ion AmpliSeq Library Preparation protocol. Template preparation, emulsion PCR and Ion Sphere Particles enrichment were performed using the Ion PGM Template OT2 200 kit (Life Technologies), according to the manufacturer’s instructions. Sequencing was performed in an Ion PGM Sequencer using an Ion 316 Chip and Ion PGM Sequencing 200 Kit v2 (Life Technologies). In total, 3 sequencing runs were carried out, with a maximum of 32 samples per run. Sequencing reads were quality-filtered and sorted according to barcodes using Torrent Suite Browser 4.0.1. On average 154,060 reads (~155 pb) were mapped against the human genome reference (hg19) per sample, of which >85% mapped to the targeted region. The mean targeted base coverage depth was 280 × (ranging from 40 to 622 × ). SNVs and indels were identified using the VariantCaller v4.0.r73742 plugin from Torrent Suite Browser. References sequences used for variant nomenclature were: DROSHA (NM_013235.4), DGCR8 (NM_022720.6), DICER1 (NM_030621.3), XPO5 (NM_020750.2), TARBP2 (NM_004178.4), CTNNB1 (NM_001904.3), WT1 (NM_000378.4), WTX (NM_152424.3), TP53 (NM_000546.5), FBXW7 (NM_018315.4) and DIS3L2 (NM_152383.4). Variants were selected based on the following criteria: (a) minimum coverage depth of 30 × ; (b) minimum variant frequency of 5%; (c) only alterations leading to amino-acid changes, splice site variants or premature stop codon were considered; (d) variants were not present in dbSNP (release #139), except to those with no minor allele frequency description ( Table 1 ). All indel and nonsense variants were selected for validation by capillary Sanger sequencing. Two DROSHA nonsense variants were also validated by allele-specific PCR (primer sequences used in this analysis are described in Supplementary Table 12 ). For missense variants, Polyphen-2 (ref. 41 ), SIFT [42] and MutationTaster [43] classification tools were used to determine the impact of amino-acid changes on protein function. Taqman low-density arrays assays TaqMan Array Human MicroRNA A Card v1.0 microfluidics cards (Life Technologies) were used to assess the miRNA profiles of 13 WT patient samples and transfected HEK293/HEK293T cells. In brief, 750 ng of total RNA was used for miRNA cDNA synthesis using the TaqMan microRNA Reverse Transcription Kit and Megaplex RT primers Human Pool A (both from Life Technologies), following the manufacturer’s protocol. cDNA products were then combined with TaqMan Universal Master Mix II with UNG (Life Technologies), and loaded into the microfluidics cards. Real-time PCR was performed on the ABI PRISM 7900HT detection system (Applied Biosystems) according to the manufacturer’s instructions. The contents of the MicroRNA A Card comprised a total of 377 unique miRNAs and three control small RNAs. In the tumours, 249 miRNAs were evaluable in at least three samples (Cq≤35) and were considered for the analysis. In the cell lines, 187 and 179 miRNAs (Cq≤35 in at least 40% of the extracts) were considered for the analyses of transiently and stably transfected cells, respectively. The array data were analysed using SDS software (Life Technologies), and miRNA levels were normalized by the average of the four replicates of the mammalian U6 reference transcript using the 2 −(delta)Cq method. For tumour samples, relative expression differences between the two groups were obtained by the ratio of the mean normalized values of the mutated to non-mutated samples. miRNAs were considered differentially expressed between the groups if the fold change was ⩾ |2| and FDR-adjusted P -value ≤0.05 (Student’s t -test). Volcano plots were generated using CLC Genomics Workbench 6.0.3 (CLCBio). Z -scores [44] of log2-transformed expression values from the differentially expressed miRNAs were used to perform unsupervised hierarchical clustering of samples. Clustering was performed with TMEV ( http://www.tm4.org/ ) using Pearson’s correlation and average linkage. For the transiently transfected cell lines, the regulation of miRNA expression of each population of cells (mock, Drosha wild-type or Drosha-E1147K) during the time course of the experiment was evaluated with STEM analysis ( http://www.cs.cmu.edu/~jernst/stem/ ), using a fold change ⩾ |2| as the parameter value (a full explanation on STEM analysis is provided at the Supplementary Methods ). For the stably transfected cells, relative expression differences between the wild-type Drosha and Drosha-E1147K cell lines were obtained by the ratio of the mean normalized values of the four passages of E1147K cells by the wild-type cells. miRNAs were considered differentially expressed between the groups if the fold change was ⩾ |2| and FDR-adjusted P -value ≤0.05 (Student’s t -test). Volcano plots were generated using CLC Genomics Workbench 6.0.3 (CLCBio). Taqman reverse-transcription qPCR The expression of eight differentially expressed and six control primary and mature miRNA pairs was assessed with TaqMan individual assays (TaqMan Pri-miRNA Assays for pri-miRNAs and TaqMan MicroRNA Assays for mature miRNAs—Life Technologies). Differentially expressed miRNAs (miR-95, miR-128a, miR-135b, miR-874, miR-876-5p, miR-126, miR-150 and miR-636) were selected based on FDR-adjusted P -value (≤0.05), fold change (≤−3.45 or ⩾ 2.0) and the availability of commercial pri-miRNA assays (taqman probes from Life Technologies). Among the non-differently expressed miRNAs, we selected six with miRNAs assays available in our lab (miR-26b, Let-7b, Let-7c, Let-7d, Let-7e and Let-7g) and used as controls. Reverse transcriptase (RT)-qPCR was performed on an ABI PRISM 7900HT detection system (Applied Biosystems) according to the manufacturer’s instructions. The relative expression levels of pri-miRNAs and miRNAs were calculated using the 2 –(delta)Cq method. Pri-miRNAs expressions were normalized by GAPDH expression and miRNAs expressions were normalized by mammalian U6. Genes were considered as differentially expressed between the groups if fold changes were ⩾ |2| and P -value ≤0.05 (Student’s t -test). Cell culture and transfection of wild-type and E1147K- DROSHA Human embryonic kidney cell lines HEK293 and HEK293T were obtained from ATCC. Cells were grown in Dulbecco’s modified Eagle’s medium (Invitrogen), supplemented with 2 mM L -glutamine, 10% bovine fetal serum, 100 U ml −1 penicillin and 100 μg ml −1 streptomycin, in a humidified atmosphere at 37 °C with 5% CO 2 . For Drosha transfection assays, we used the pcDNA4/TO/cmycDrosha plasmid [27] (Addgene #10828) containing the wild-type Drosha sequence. To obtain an E1147K DROSHA -expressing plasmid, we performed site-directed mutagenesis using the QuikChange II-XL Site-Directed Mutagenesis Kit (Agilent Technologies). PCR products were cloned into XL10-Gold Ultracompetent Cells using heat-shock transformation. The presence of the mutation was confirmed on selected clone inserts by capillary Sanger sequencing of the flanking region. HEK293 cells were transfected in six-well plates at 90% confluent layer with 2.5 μg of wild-type DROSHA , E1147K DROSHA and mock plasmids using Lipofectamine LTX Reagent (Life Technologies), according to the manufacturer’s instructions. The transient transfections were performed twice in a 72-h interval, and total RNA was extracted 48 h after the first transfection, 48 h after the second transfection and 72 h after the second transfection. HEK293T cells were stably transfected using the same conditions described for HEK293. After 24 h of transfection, the medium was replaced with medium containing Zeocin 150 μg ml −1 (Invitrogen). Selection was performed for 15 days. Western blot Western blotting was performed to detect the expression of transfected wild-type and E1147K DROSHA in HEK293 and HEK293T cell lines. Cell pellets were diluted in RIPA buffer with phosphatase inhibitor cocktail 3 (1:100, Sigma-Aldrich) and protease inhibitor cocktail (1:100, Sigma), and lysed by temperature change (dry ice and 37 °C repeated 10 × ). Protein concentration was quantified using the QuantiPRO BCA assay kit (Sigma-Aldrich), loaded onto an SDS-PAGE gel (10%) and transferred onto polyvinylidene difluoride membrane. The blots were probed with anti-myc-HRP (1:5,000, Invitrogen), anti-Drosha (rabbit monoclonal, 1:1,000, Cell Signaling) and anti-GAPDH (mouse polyclonal, 1:1,000, Invitrogen) at 4 °C overnight and subsequently incubated with horseradish peroxidase-conjugated secondary antibody (1:3,000). Signals were visualized using ECL Substrates (Millipore) and captured with UVItec Alliance 4.7 (UVItec) ( Supplementary Figs 5b, 7b and 8 ). For quantification of proteins bands, densitometry was performed with ImageJ 1.4 ( http://imagej.software.informer.com/1.4/ ). SYBR Green qPCR RT–qPCR was performed to confirm the expression of transfected wild-type and E1147K DROSHA in HEK293/HEK293T cell lines. Briefly, 1 μg total RNA was converted into cDNA in the presence of SuperScript III RT (Invitrogen) and oligo(dT)18. Reactions were performed using cDNA converted from 10 ng of RNA, 250 nM of each primer and 1 × SYBR Green PCR Master Mix (Life Technologies) in a total volume of 20 μl. Primers used for DROSHA were as previously described [45] (forward: 5′-TAGGCTGTGGGAAAGGACCAAG-3′; reverse: 5′-GTTCGATGAACCGCTTCTGATG-3′). ACTB and GAPDH were used for data normalization. Mock transfected cells were used as a calibrator and relative fold changes were calculated using the 2 –[delta][delta]Cq method ( Supplementary Figs 5c and 7c ). How to cite this article: Torrezan, G. T. et al . Recurrent somatic mutation in DROSHA induces microRNA profile changes in Wilms tumour. Nat. Commun. 5:4039 doi: 10.1038/ncomms5039 (2014). Accession codes: Exome sequence data has been deposited in the European Nucleotide Archive, hosted by the European Bioinformatics Institute, under the accession code PRJEB6113 .